Proteome adaptation in cell reprogramming proceeds via distinct transcriptional networks The ectopic expression of Oct4, Klf4, c-Myc and Sox2 (OKMS) transcription factors allows reprogramming of somatic cells into induced pluripotent stem cells (iPSCs). The reprogramming process, which involves a complex network of molecular events, is not yet fully characterized. Here we perform a quantitative mass spectrometry-based analysis to probe in-depth dynamic proteome changes during somatic cell reprogramming. Our data reveal defined waves of proteome resetting, with the first wave occurring 48 h after the activation of the reprogramming transgenes and involving specific biological processes linked to the c-Myc transcriptional network. A second wave of proteome reorganization occurs in a later stage of reprogramming, where we characterize the proteome of two distinct pluripotent cellular populations. In addition, the overlay of our proteome resource with parallel generated -omics data is explored to identify post-transcriptionally regulated proteins involved in key steps during reprogramming. The expression of a cocktail of defined transcription factors is a well-known strategy to reprogram somatic mammalian cells to a pluripotent state named induced pluripotent stem cells (iPSCs) [1] Several studies have demonstrated that iPSCs resemble their embryo-derived counterpart embryonic stem cells (ESCs) both at the functional and molecular levels [2] , [3] , [4] , [5] , [6] , [7] , [8] , [9] , [10] , [11] , [12] , [13] , [14] . Owing to their properties, the development of iPSCs technology has a huge impact both in basic research and clinical applications. To date, various somatic cell types from diverse adult tissues (that is, endoderm, mesoderm and ectoderm origins) have been successfully reprogrammed to iPSCs [1] , [15] , [16] , [17] , [18] . However, the overall frequency in which the transition to pluripotency occurs is typically low (<1%) and requires 1–3 weeks of factors expression. Nevertheless, as shown by others, the kinetics and efficiency of this process can be manipulated by either controlling the expression of specific molecular mediators [19] , [20] , [21] , [22] or through the use of chemical compounds [23] , [24] . Thus, understanding the molecular mechanisms involved in cellular reprogramming may enable the improvement of the efficiency of this process. The molecular characterization of intermediate cellular states occurring during the reprogramming process has so far been poorly addressed largely due to (i) its extended latency, (ii) with only a small subset of the starting cells becoming pluripotent and (iii) leading to cellular heterogeneity. To overcome this limitation, secondary expression systems with inducible polycistronic constructs have been used [25] , [26] , [27] . These studies provide evidence that reprogramming is a multistep process in which pluripotency is acquired via step-wise transitions through defined transcriptional states [28] , involving the early induction of cellular proliferation and downregulation of differentiation markers, followed by a mesenchymal-to-epithelial transition (MET) [29] , [30] . Although these reports represent an invaluable source of knowledge to decipher the molecular mechanisms governing the different phases of reprogramming, the study of the dynamic changes at the proteome level is not yet fully explored. It has been shown that different levels of gene expression regulation (that is, epigenetic marks, mRNA expression and non-coding RNAs) have a synergic effect on determining the final levels of proteins [31] . Genome-wide profiling of the proteome can be best approached by mass spectrometry (MS)-based techniques, which allow the identification and quantification of several thousands of proteins [32] , [33] . As far as iPSCs are concerned, MS-based profiling has been used to compare the proteomes of human iPS and ES cells [34] , [35] . Recently, protein expression changes during reprogramming have been investigated revealing the occurrence of highly coordinated proteomic changes in this process [36] . However, such analysis included five time points, which may have limited the chance to capture additional stage-specific events. Moreover, the use of pre-selected cell populations ‘on route’ to pluripotency (that is, using specific markers such as SSEA1, Thy-1 and Oct4-GFP) might neglect the existence of additional mechanisms arising simultaneously in reprogramming cells. Indeed, we have demonstrated that ESC-like cells are not the only pluripotent outcome of the reprogramming process [37] . We have identified a new category of steady-state pluripotent cells (F-class), which can appear when the reprogramming factors are expressed at high levels [37] . Here, we use our transposon-based secondary reprogramming system [27] to quantitatively probe, at an unprecedented depth, the proteome changes of reprogramming cells in 13 different time points. By using a dual transgene expression scheme, we isolate two different cellular populations established in the late phase of reprogramming (F-class and ESC-like cells) and demonstrate that they exhibit unique proteomic features. As part of a multi-omics joint consortium [37] , [38] , [39] , [40] , we have also investigated the presence of post-transcriptional mechanisms that might tune final protein levels. To profile proteome changes at different stages of somatic cell reprogramming, we used our secondary mouse embryonic fibroblast (2°MEF) cell line (1B), generated by a doxycycline (dox)-inducible piggyBac transposon-based transgene delivery system [27] . A modulated transgene expression scheme was used to model cell reprogramming towards the fuzzy colony-forming state (F-class) [37] and the ESC-like state. Briefly, after 16 days of transgene expression, induced by high concentrations of doxycyclin (high dox=1,500 ng ml −1 ), the cellular population is dominated by cells representing the F-class state. Attenuated transgene expression obtained by dropping the dox concentration 300-fold to 5 ng ml −1 at day 8, facilitated the transition of reprogramming cells to the ESC-like state [38] . Although the Nanog + F-class cells share some properties with the ESC-like state (immortality, self-renewal, teratoma formation and in vitro differentiation capability), they differ with respect to cell morphology, transgene dependence and ability to integrate into pre-implantation embryos and to form chimaeras [37] . A total of 13 samples, representing the temporal course of reprogramming, were subjected to in-depth quantitative proteomic analysis ( Fig. 1 ). We analysed the precursor 2°MEF, six intermediate time points (day 2, 5, 8, 11, 16 and 18) at high-dox concentrations (termed D2 H, D5 H, D8 H, D11 H, D16 H and D18 H) and three intermediate time points (day 16 and 21) collected after reducing the doxycyclin concentration (low dox) starting from day 8 (termed D16 L, D21 L, D21 Ø). In addition, we analysed the secondary iPSCs (termed 2°iPSC), primary iPSCs (termed 1°iPSC) and Rosa26-rtTA transgenic ESCs, which represent the ESC-like pluripotency (termed ESC). By using a combination of isobaric peptide labelling, strong cation exchange (SCX) chromatography and high-resolution tandem mass spectrometry (LC-MS/MS) analysis, we identified a total of 7,250 proteins and quantified 4,454 of those in all the samples analysed ( Supplementary Figs 1 and 2 and Supplementary Data 1 ). Importantly, 55% of the proteins quantified ( n =2,452) changed more than twofold in at least one of the samples (when compared with the 2°MEF), indicating that the dox-induced OKMS expression results in widespread proteome changes. 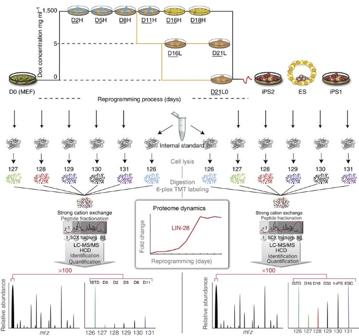Figure 1: Schematic overview of the experimental proteomics workflow. Treatment of 1B 2°MEF with doxycycline (1,500 ng ml−1)-induced OKMS expression and initiated reprogramming, which was monitored at five consecutive time points (D2H,D5H,D8H,D11H,D16H andD18H). Modulation of transgene expression was induced by dropping the dox concentration to 5 ng ml−1after 8 days, whereafter three samples were profiled:D16L,D21L andD21Ø (in the latter sample, doxycycline was completely removed on day 14). In addition, the original 2°MEFs, a Rosa rtTA ESC line, as well as the primary and secondary iPSCs (1°iPSC and 2°iPSC) were included in our quantitative proteome analysis. All the 13 collected samples were processed for proteomic analysis (lysis, proteolysis, TMT-based isotope labelling) and grouped in three mixtures before SCX fractionation and LC-MS/MS analysis, whereby each mixture included a common internal standard (ISTD). Temporal expression profiles were obtained using differential quantification versus this common ISTD. Figure 1: Schematic overview of the experimental proteomics workflow. Treatment of 1B 2°MEF with doxycycline (1,500 ng ml −1 )-induced OKMS expression and initiated reprogramming, which was monitored at five consecutive time points ( D2 H, D5 H, D8 H, D11 H, D16 H and D18 H). Modulation of transgene expression was induced by dropping the dox concentration to 5 ng ml −1 after 8 days, whereafter three samples were profiled: D16 L, D21 L and D21 Ø (in the latter sample, doxycycline was completely removed on day 14). In addition, the original 2°MEFs, a Rosa rtTA ESC line, as well as the primary and secondary iPSCs (1°iPSC and 2°iPSC) were included in our quantitative proteome analysis. All the 13 collected samples were processed for proteomic analysis (lysis, proteolysis, TMT-based isotope labelling) and grouped in three mixtures before SCX fractionation and LC-MS/MS analysis, whereby each mixture included a common internal standard (ISTD). Temporal expression profiles were obtained using differential quantification versus this common ISTD. Full size image Using this subset of 2,452 differential proteins, we first examined the global correlation over all the samples ( Fig. 2a , Supplementary Data 2 ). This analysis revealed at least six distinct groups, (a) the precursor 2°MEF, (b) the first high-dox sample ( D2 H), (c) the further transient high-dox cells ( D5 H– D11 H), (d) F-class state (represented by D16 H and D18 H), (e) the low-dox ( D16 L, D21 L, D21 Ø) samples and (f) 1°iPSC, 2°iPSC and ESC. Two days following dox-induced OKMS protein expression, the proteome was already very distinct from the original fibroblast proteome. After that, a distinctive step-wise temporal progression of the reprogramming process was evident in the high-dox samples, where D5 H cells displayed a high similarity with the subsequent time points D8 H and partially with D11 H. Notably, the dynamic changes observed from D2 H until D11 H turned into a stable proteome state at D16 H and D18 H. Cells at these latter two time points were almost indistinguishable at the proteome level and represent the aforementioned F-class cells ( Fig. 2a ). Notably, these F-class cells represent a stable state and do not turn into an ESC-like state even after 2 additional weeks of high-dox treatment [37] . However, following the reduction of transgene expression, the population of reprogramming cells morphologically resembled ESCs [38] . In agreement with these findings, our proteomic data show that the low-dox cells ( D16 L, D21 L and D21 Ø) share not only a high proteome correlation between each other, but also with the ESC-like state samples ( Fig. 2a ). Next, we investigated the proteomic behaviour of genes related to pluripotency and self-renewal as reported in the Plurinet resource [41] . From the 282 Plurinet genes, our data contained quantitative measurements for 129 proteins that we used to assess the correlation between the different cell states. This focused analysis revealed a lower correlation for all the reprogramming cells with the ESC-like group, compared with the global proteome analysis ( Fig. 2a,b ), which means that none of these cells undergo a full activation of the pluripotency network. Moreover, weak Plurinet-based correlation changes between the 2°MEF and the cells exposed to high-dox conditions is evident, while low-dox cells are clearly distinct ( Fig. 2b ). When compared with ESC, the correlation of 2°MEF and high-dox samples is constantly low. In contrast, attenuated transgene expression led to a substantial increase in similarity with the ESC-like state ( Fig. 2c ). 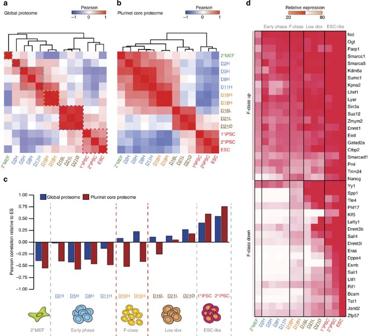Figure 2: Proteome adaptation occurs in waves during somatic cellular reprogramming. Pearson correlation values were calculated for all 13 samples analysed on the basis of (a) all proteins showing >twofold change relative to 2°MEF levels (n=2,445) and (b) all proteins belonging to the Plurinet core-proteome (n=129). (c) Bar chart of the calculated Pearson correlation values relative to ESCs for each of the samples analysed. Global proteome and Plurinet core-proteome Pearson values are shown in blue and red, respectively. (d) Differential expression of specific Plurinet core-proteome proteins, relative to ESCs, in F-class, low-dox and ESC-like samples. Figure 2: Proteome adaptation occurs in waves during somatic cellular reprogramming. Pearson correlation values were calculated for all 13 samples analysed on the basis of ( a ) all proteins showing >twofold change relative to 2°MEF levels ( n =2,445) and ( b ) all proteins belonging to the Plurinet core-proteome ( n =129). ( c ) Bar chart of the calculated Pearson correlation values relative to ESCs for each of the samples analysed. Global proteome and Plurinet core-proteome Pearson values are shown in blue and red, respectively. ( d ) Differential expression of specific Plurinet core-proteome proteins, relative to ESCs, in F-class, low-dox and ESC-like samples. Full size image Intrigued by these findings, we investigated which Plurinet proteins exhibited differential expression between F-class, low-dox and ESC-like cells. This analysis revealed that proteins involved in nuclear processes (for example, Ncl, Lyar, Parp1, Kpna2) and chromatin architecture establishment (for example, Uhfr1, Kdm6a, Eed, Suz12, Smarca5, Smarcad1, Smarcc1), and also Nanog, were expressed at comparable upregulated levels within both pluripotent cell populations ( Fig. 2d ). However, in F-class cells, several pluripotency markers (for example, Sall4, Utf1, Dppa4, Lefty and Esrrb) were less abundant than both the low-dox and ESC-like cells ( Fig. 2d ) (a finding supported by transcriptomic analyses performed in parallel [38] ). Recently, it has been proposed that iPSCs may retain an epigenetic memory of their parental cells [42] , [43] . Using our reprogramming system, we have observed in F-class that the low expression of many pluripotency genes is associated with 5-methylcytosine and H3K27me3 inhibitory marks [37] , [38] , [40] . In the current data set, we found reduced levels of proteins involved in DNA methylation (for example, Dnmt3b, Dnmt3l, Zfp57, Tet1), telomeres binding (for example, Rif1, Terf1) and other epigenetic-based transcriptional regulators (for example, Pml, Phf17, Jarid2 and Yy1) in F-class cells. Notably, Tet1 has been shown to replace Oct4 and initiate somatic cell reprogramming in conjunction with Sox2, Klf4 and c-Myc [44] . Moreover, although some proteins involved in epigenetic control of gene expression (that is, Suz12 and Eed subunits of the Polycomb complex 2) were highly expressed by F-class, low-dox and ESC-like cells, there were two important modulators of this complex, Jarid2 and Yy1 (refs 45 , 46 ), present at a lower level specifically in F-class cells ( Fig. 2d ). The systems-level nature of our analyses allowed us to investigate whether the reprogramming process could be to a certain extent regulated post-transcriptionally. We compared our protein measurements with mRNA-seq data derived in parallel [38] . Throughout all time points, we observed a reasonable, albeit not perfect, correlation between mRNA and protein changes (Pearson’s correlatio n ~0.5; Fig. 3a ). However, the low-dox samples exhibited a substantial lower correlation (Pearson’s ~0.25). We then selected arbitrarily the uppermost 1,275 genes, for which protein and mRNA showed poor correlation (see Methods) in F-class, ESC-like and low-dox cells ( Fig. 3b ) where the poor correlation was particularly evident. We next categorized these 1,275 genes in four subsets on the basis of whether protein levels displayed up- or downregulation, but no change in mRNA and vice versa, and probed if the genes in any of these subsets were enriched in particular GO terms (see Methods). As shown in Fig. 3c , the data suggest that, particularly in low-dox cells, post-transcriptional regulatory mechanisms control the expression at the protein level of genes involved in cellular adhesion (for example, remodelling of epithelial adherens junctions, integrin and paxillin signalling), oestrogen and androgen signalling and mitochondrial function. The observed downregulation of these proteins may be controlled more intensely by ubiquitin-dependent degradation rather than translational control. 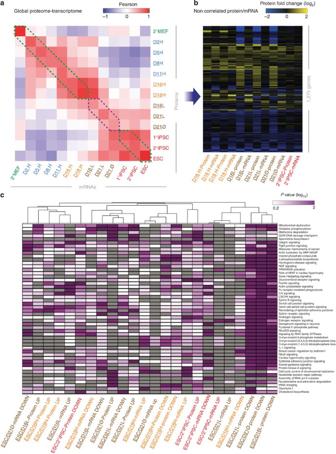Figure 3: Identification of stage-specific post-transcriptional mechanisms. (a) Pair-wise comparisons between mRNA and protein levels (n=2,424). (b) Heat-map of protein and mRNA levels of the top-most poor correlating 1,275 genes for theD16H,D18H,D16L,D21L,D21Ø and 2°iPSC cells. Their relative expression level is always compared with ESC (Log2ratio). (c) The most enriched pathways are displayed as a heat-map, based on their Log10of thePvalue, and identified specific enrichment of non-correlating genes in low-dox cells. Figure 3: Identification of stage-specific post-transcriptional mechanisms. ( a ) Pair-wise comparisons between mRNA and protein levels ( n =2,424). ( b ) Heat-map of protein and mRNA levels of the top-most poor correlating 1,275 genes for the D16 H, D18 H, D16 L, D21 L, D21 Ø and 2°iPSC cells. Their relative expression level is always compared with ESC (Log 2 ratio). ( c ) The most enriched pathways are displayed as a heat-map, based on their Log 10 of the P value, and identified specific enrichment of non-correlating genes in low-dox cells. Full size image To draw an unbiased picture of the dynamic proteomic changes occurring at different phases of reprogramming, we next clustered the 2,452 differential proteins on the basis of their time course expression during the reprogramming process (from 2°MEF to 2°iPSC) into nine distinct profiles ( Fig. 4a ). For figure legibility and better show of the temporal sequence of the reprogramming process, we did not include 1°iPSC and ESC samples in such analysis, as these samples show similar proteome profiles with 2°iPSC ( Fig. 2a ). We subsequently investigated whether the proteins within a cluster shared functionality. These analyses revealed the involvement of specific molecular processes in certain phases of the reprogramming process. For instance, early proteomic changes showed a highly coordinated activation (cluster 1 and 7) of the cellular machinery necessary to sustain increased cellular kinetics (proteins involved in cell cycle control, cellular proliferation, metabolism and energy production) and the refined tuning of expression programs (RNA processing, gene expression, nucleolar proteins) ( Fig. 5 and Supplementary Fig. 3a,b ). We also found that fibroblasts rapidly lose their cellular identity by downregulating mesenchymal markers (clusters 3 and 8 Fig. 4b ), as well as proteins related to glycosylation, vesicle transport, extracellular matrix and energy reserve metabolism ( Fig. 5 and Supplementary Fig. 3b ). Interestingly, interrogation of available ChIP-seq data [47] revealed that the first wave of proteome resetting is strongly enriched for target genes of c-Myc, Kdm5b and Jarid2a pointing out these transcription factors as having key roles in these early events ( Fig. 5 and Supplementary Fig. 4 ). These findings are in agreement with recent gene expression and proteomic analyses in a different secondary reprogramming design restricted toward ESC-like pluripotency [28] , [36] . 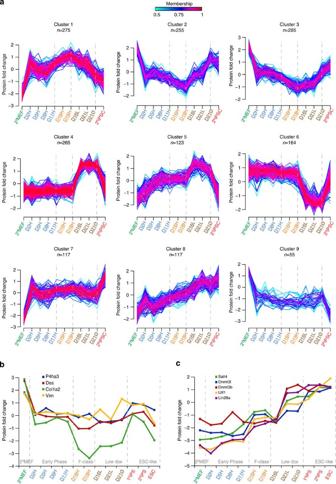Figure 4: Clustering of proteome expression profiles during reprogramming. (a) Proteins quantified across the whole sample set and showing a fold change higher than two were subjected to unsupervised clustering with the Fuzzy c-means algorithm. Nine distinct patterns of dynamic changes could be classified, whereby the number of proteins included in each cluster is indicated. Colour-coded membership represents how well a single protein pattern fits with the general profile of the cluster. (b) Expression profiles of individual well-known fibroblast-associated proteins. (c) Expression profiles of defined individual pluripotency markers. Figure 4: Clustering of proteome expression profiles during reprogramming. ( a ) Proteins quantified across the whole sample set and showing a fold change higher than two were subjected to unsupervised clustering with the Fuzzy c-means algorithm. Nine distinct patterns of dynamic changes could be classified, whereby the number of proteins included in each cluster is indicated. Colour-coded membership represents how well a single protein pattern fits with the general profile of the cluster. ( b ) Expression profiles of individual well-known fibroblast-associated proteins. ( c ) Expression profiles of defined individual pluripotency markers. 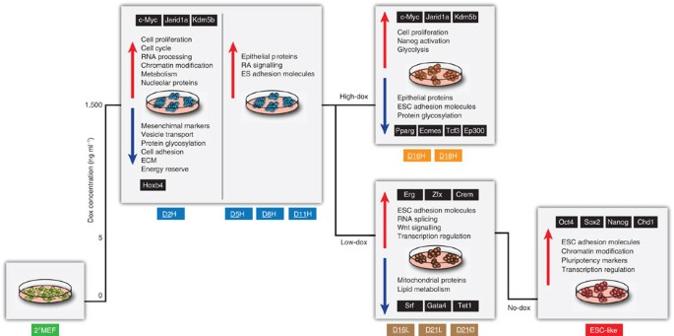Figure 5: Model describing the observed proteome dynamics during key steps in the reprogramming. Summary of the most relevant cellular states occurring during the reprogramming process depicted by (i) main proteomic features concerning the enriched GO terms and KEGG pathways and (ii) TFs predicted to control a set of protein targets differentially expressed in the different steps of reprogramming. GO terms, KEGG pathways and TFs relative to upregulated and downregulated proteins are shown in red and blue, respectively. Full size image Figure 5: Model describing the observed proteome dynamics during key steps in the reprogramming. Summary of the most relevant cellular states occurring during the reprogramming process depicted by (i) main proteomic features concerning the enriched GO terms and KEGG pathways and (ii) TFs predicted to control a set of protein targets differentially expressed in the different steps of reprogramming. GO terms, KEGG pathways and TFs relative to upregulated and downregulated proteins are shown in red and blue, respectively. Full size image To further investigate causative or descriptive markers in the co-occurring pluripotency routes, we focused on proteome adaptation observed at the intermediate phase. Subtle changes occur from D5 H until D11 H, whereby cells exhibit an increased level of epithelial proteins, retinoic acid signalling and ESC-specific adhesion molecules ( Supplementary Fig. 5 ), consistent with the MET that is required as one of the key processes during fibroblast reprogramming [29] , [30] . In the late reprogramming phase, more prominent proteome changes are observed in both F-class and low-dox cells. F-class cells are uniquely characterized by a coordinated loss of epithelial and ESC-specific adhesion proteins (with the exception of Epcam) compared with D5 H– D11 H, low-dox and ESC-like samples ( Supplementary Fig. 5a,b ). Instead, proteins exhibiting their maximum expression in F-class cells are associated with metabolism and cellular proliferation (cluster 1) and are mainly regulated by the c-Myc transcriptional network ( Fig. 5 and Supplementary Fig. 4 ). The fact that high-dox conditions lead to a reprogramming path characterized by an early MET, followed by an EMT transition and an increase in cellular metabolism is further reflected by miRNAs analysis [39] , where an altered expression of pro-MET, pro-EMT and mitochondrial RNA is observed in the same set of samples. It is intriguing that F-class state may be linked to the activation of specific expression programs occurring when the cells have acquired epithelial traits. Coincidently with this phase of reprogramming, we noticed an early and transient upregulation of proteins involved in retinoic acid (RA) signalling (Rbp1, Aldh1a1and Gprc5a) ( Supplementary Fig. 5c ). Notably, opposing effects of RA on cell proliferation correlates to the level of two RA binding proteins, Crabp2 and Fabp5 (ref. 48 ). In cells characterized by a high Crabp2/Fabp5 ratio, RA signalling results in the activation of RAR nuclear receptors and exhibit a proapoptotic activity, whereas high level of Fabp5 protein results in the activation of the nuclear receptors Pparβ/δ, promoting cell survival In reprogramming cells, these two RA binding proteins showed a sequential upregulation, with Crabp2 being upregulated only in D8 H and D11 H and Fabp5 in F-class cells ( Supplementary Fig. 5c,d ), possibly representing one of the mechanisms involved in the establishment of the F-class cell type [21] . Cluster 8 contains proteins that demonstrate the highest expression in the 2°iPSC ( Fig. 4a ), with limited activation in F-class cells. Several well-known ES cells markers belong to this cluster ( Fig. 4c ). Functional analysis revealed a strong enrichment for proteins involved in DNA replication, transcription regulation, as well as chromatin modification ( Fig. 5 and Supplementary Fig. 3a,b ). These results confirmed, at the global proteome level, our finding that low-dox cells closely resemble the expression level of proteins upregulated in ESC-like state (see Plurinet analysis in Fig. 2d ). Of note, we also found that the significant proportion of proteins highly expressed in ESC-like cells are controlled transcriptionally by Sox2, Oct4, Nanog and Chd1 ( Fig. 5 and Supplementary Fig. 4 ). To define the common molecular imprint between F-class and ESC-like cells controlled by these key transcription factors, we first selected the known target proteins of Nanog, Oct4 and Sox2 (ref. 47 ) found to be upregulated in 2°iPSC and ESC ( Fig. 6a , Supplementary Data 3 ). Next, we defined the specific subset of protein targets, which remain silent or partially active (upregulated compared with 2°MEF and downregulated compared with ESC-like) in F-class cells ( Fig. 6a ) and monitored the dynamic activation of these targets across the whole reprogramming window ( Fig. 6b ). Notably, the partial activation of the ESC-like pluripotency network in F-class cells seems to be sufficient to confer them pluripotent traits, whereby all three germ layers can be generated in a teratoma-forming assay [37] . 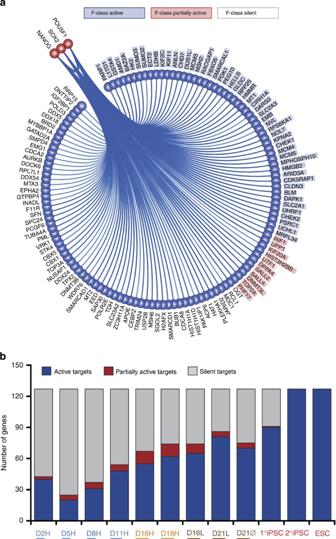Figure 6: The pluripotency protein network is more extensive in ESCs and iPSCs than in F-class (high-dox) cells. (a) Nanog, Oct4 and Sox2 (red dots) transcriptional network active in ES-like cells. Blue dots represent protein targets upregulated in ES-like cells. The subset of protein targets, which are either active (blue highlights) or partially active (red highlights) in F-class cells are distinguished by the subset of protein targets, which are silent in this cell type (no highlights). (b) Dynamic activation of Nanog, Oct4 and Sox2 transcriptional network across the reprogramming process (bars representing active targets are in blue, partially active targets in red and silent targets in grey). Figure 6: The pluripotency protein network is more extensive in ESCs and iPSCs than in F-class (high-dox) cells. ( a ) Nanog, Oct4 and Sox2 (red dots) transcriptional network active in ES-like cells. Blue dots represent protein targets upregulated in ES-like cells. The subset of protein targets, which are either active (blue highlights) or partially active (red highlights) in F-class cells are distinguished by the subset of protein targets, which are silent in this cell type (no highlights). ( b ) Dynamic activation of Nanog, Oct4 and Sox2 transcriptional network across the reprogramming process (bars representing active targets are in blue, partially active targets in red and silent targets in grey). Full size image Although the low-dox cells closely resemble the ESC-like state in general terms, they also exhibit a set of proteins with abundances significantly different from the 2°iPSC ( Fig. 4 , clusters 4 and 6). These proteins may point to mechanisms involved in the stabilization of these cells towards a mature ES-like phenotype ( Supplementary Fig. 3 ). Numerous proteins involved in post-transcriptional (mRNA splicing) and post-translational (ubiquitin-mediated proteolysis) regulation were grouped in cluster 4. Also, several proteins known to activate either the canonical and non-canonical Wnt pathway were present in the same cluster, which is in agreement with the upregulation of beta-catenin in low-dox cells compared with F-class ( Supplementary Fig. 5 ). Predicted upstream TFs for the members of this cluster included the chromatin modifier enzyme Crem and Erg, as well as Zfx, known to control self-renewal [49] . Our proteomics data, in conjunction with the in-parallel-generated complementary -omics data [38] , represents a unique resource to further study the molecular mechanisms of the reprogramming process. To the best of our knowledge, this analysis represents the most comprehensive proteomic profiling of the reprogramming process, both in terms of its temporal resolution and its cellular outcomes characterization. We confirmed the processes involved in the early transition recently published in gene expression and proteomic analyses [28] , [36] , suggesting that they represent well-defined features of the early step of reprogramming regardless of the system used to generate iPSCs or the cellular subpopulation selected for the analysis. In addition, we were able to define and isolate two different reprogramming routes leading to the F-class [37] and ESC-like state through a dual transgene expression scheme ( Fig. 1 ). Our analyses indeed revealed a second wave of global proteome adaptation occurring in two distinct pluripotent cellular populations both of which involved activation of Nanog but showed differences in adhesion properties, cell metabolism and gene expression control. Therefore, our experimental design and data set represent an ideal system to capture and characterize multiple routes leading to pluripotency. Cell culture and secondary reprogramming ESCs and iPSCs were cultured in 5% CO 2 at 37 °C on irradiated MEFs in DMEM containing 15% FCS, leukemia-inhibiting factor, penicillin/streptomycin, L-glutamine, nonessential amino acids, sodium pyruvate and 2-mercaptoethanol. 1B 1° iPS cells were aggregated with tetraploid host embryos as described [27] and MEFs established from E13.5 embryos. Fibroblasts were expanded to passage three with one billion fibroblasts forming the basis of the reprogramming system. Cell reprogramming was induced by exposure to 1,500 ng ml −1 doxycycline (dox). Reprogramming cells were maintained as two parallel cultures passaged on alternate days (three day intervals), to ensure that biological samples were consistently collected 48 h after passaging. Cell reprogramming was induced by exposure to 1,500 ng ml −1 doxycycline (dox). Reprogramming cells were maintained as two parallel cultures passaged on alternate days (three day intervals), to ensure that biological samples were consistently collected 48 h after passaging. High doxycycline cell samples were collected at days 0, 2, 5, 8, 11, 16 and 18 ( D2 H, D5 H, D8 H, D11 H, D16 H, D18 H). A subculture of the reprogramming cells was established from day 19 and cultured in the absence of dox, to develop a factor-independent 2° iPS cell line by day 30 (2°iPSC). Low-dox samples were maintained from day 8 to day 14 cells in 5 ng dox. At day 14, the culture was diverged in two with some of the cells being cultured until day 21 in the absence of dox ( D21 Ø) and the remainder were cultured in 5 ng ml −1 of dox and collected at day 16 ( D16 L) and day 21 ( D21 L). Rosa26-rtTA ESCs and 1B 1 o iPSCs were collected as controls. Sample preparation for MS analysis Secondary MEFs, primary and secondary miPSCs, mESCs, six intermediate reprogramming time points in high-dox conditions ( D2 H, D5 H, D8 H, D11 H, D16 H and D18 H) and three intermediate reprogramming time points in low-dox conditions ( D16 L, D21 L, D21 Ø) were collected by centrifugation at 2,500 g for 10 min at 4 °C. Cell lysis was performed in a buffer containing 8 M urea in a solution of 100 mM triethyl ammonium bicarbonate (Fluka), pH 8.2, with protease and phosphatase inhibitors (Roche). Proteins (~1 mg) were first reduced/alkylated and digested for 4 h with Lys-C. The mixture was then diluted fourfold to 2 M urea and digested overnight with sequencing-grade trypsin (Promega) in substrate/enzyme ratio of 50:1 (w/w). Digestion was quenched by acidification with formic acid (FA) (final concentration 10%). Resulting peptides were subsequently desalted by solid phase extraction (Sep-pack Vac C18 cartridges, Waters), vacuum dried and then re-suspended in triethyl ammonium bicarbonate buffer 100 mM to a final concentration of ~1 mg ml −1 . An aliquot of 100 μg of each sample was chemically labelled with Tandem Mass Tag (TMT) reagents [50] (Thermo Fisher) according to the manufacturer’s instructions. To accommodate all the 13 samples in the analysis, three TMT mixtures were created. Basically, ‘mix1’ contained a set of five different samples mixed in a 1:1 ratio (secondary MEFs and day 2, 5, 8 and 11). ‘Mix2’ contained the other set of samples mixed in a 1:1 ratio ( D16 H, D18 H, ESC, 1°iPSCs and 2°iPSCs). ‘Mix3’ contains the low-dox samples mixed in a 1:1 ratio. An internal standard consisting of a mixture in a 1:1 ratio of all the samples included in mix1 and 2 (labelled with TMT reagent 126) was also included in ‘Mix1’, ‘Mix2’ and ‘Mix3’. This internal standard was used for data normalization and integration of both data sets ( Supplementary Fig.1 ). Before the mass spectrometric analysis, both the TMT-labelled peptides mixtures were fractionated as described elsewhere [51] . The SCX system consisted of an Agilent 1200 HPLC system (Agilent Technologies, Waldbronn, Germany) with one C18 Opti-Lynx (Optimized Technologies, OR) trapping cartridges and a Zorbax BioSCX-Series II column (0.8-mm inner diameter, 50-mm length, 3.5 microms particle size). The labelled peptides were dissolved in 10% FA and loaded onto the trap columns at 100 μl min −1 and subsequently eluted onto the SCX column with 80% acetonitrile (ACN; Biosolve, The Netherlands) and 0.05% FA. SCX solvent A consists of 0.05% formic acid in 20% ACN, while solvent B was 0.05% formic acid, 0.5 M NaCl in 20% ACN. The SCX salt gradient is as follows: 0–0.01 min (0–2% B); 0.01–8.01 min (2–3% B); 8.01–14.01 min (3–8% B); 14.01–28 min (8–20% B); 28–38 min (20–40% B); 38–48 min (40–90% B); 48–54 min (90% B); 54–60 min (0% B). A total of 50 SCX fractions (1 min each, that is, 40 μl elution volume) were collected and used for subsequent LC-MS/MS analysis. Mass spectrometric analysis We performed nanoflow LC-MS/MS using an LTQ-Orbitrap Velos mass spectrometer (Thermo Electron, Bremen, Germany) coupled to an Agilent 1200 HPLC system (Agilent Technologies). SCX fractions were dried, reconstituted in 10% FA and delivered to a trap column (ReproSil C18, (Dr Maisch GmbH, Ammerbuch, Germany); 20 mm × 100 μm inner diameter, packed in-house) at 5 μl min −1 in 100% solvent A (0.1 M acetic acid in water). Next, peptides eluted from the trap column onto an analytical column (ReproSil-Pur C18-AQ (Dr Maisch GmbH, Ammerbuch, Germany); 40 cm length, 50 μm inner diameter, packed in-house) at ~100 nl min −1 in a 90 min or 3 h gradient from 0–40% solvent B (0.1 M acetic acid in 8:2 (v/v) ACN/water). The eluent was sprayed via distal coated emitter tips butt-connected to the analytical column. The mass spectrometer was operated in data-dependent mode, automatically switching between MS and MS/MS. Full-scan MS spectra (from m / z 350–1,500) were acquired in the Orbitrap with a resolution of 30,000 FHMW at 400 m / z after accumulation to target value of 500,000 in the linear ion trap (maximum injection time was 250 ms). After the survey scans, the 10 most intense precursor ions at a threshold above 5,000 were selected for MS/MS with an isolation width of 1.2 Da after accumulation to a target value of 30,000 (maximum injection time was 50 ms). Peptide fragmentation was carried out by using higher-energy collisional dissociation with an activation time of 0.1 ms and a normalized collision energy of 45%. Fragment ions analysis was performed in the Orbitrap with a resolution of 7,500 FHMW and a low mass cut-off setting of 100 m / z . Each SCX fraction was analysed at least in triplicate, with a 90 min or 3 h LC gradient, depending on their complexity. Data processing MS raw data were processed with Proteome Discoverer (version 1.3, Thermo Electron). Basically, peptide identification was performed with Mascot 2.3 (Matrix Science) against a concatenated forward-decoy UniPROT database supplemented with all the frequently observed contaminants in MS (version 5.62). The following parameters were used: 50 p.p.m. precursor mass tolerance, 0.02 Da fragment ion tolerance, up to two missed cleavages, carbamidomethyl cysteine as fixed modification, oxidized methionine and TMT modification on amino (N)-term and Lysine as variable modifications. Finally, we performed a deconvolution of the high-resolution MS2 spectra, by which all the fragment ions isotopic distributions were converted to an m / z value corresponding to the monoisotopic single charge. Reporter ion-based quantification method was chosen in Proteome Discoverer, with the following requirements for reporter ion integration in the MS2 spectra; mass accuracy of maximum 20 p.p.m., peptide ratio maximum limit 100. To minimize ratio distortion due to the presence of more than one peptide species within the precursor ion isolation width, we also reject the quantification of MS/MS spectra having a co-isolation higher than 30%. Finally, results were filtered using the following criteria: (i) mass deviations of ±5 p.p.m., (ii) Mascot Ion Score of at least 25, (iii) a minimum of seven amino-acid residues per peptide and (iv) position rank 1 in Mascot search. As a result, we obtained peptide FDRs [52] below 1% for all of the three peptide mixtures analysed ( Supplementary Data 1 ). Finally, peptide ratios were Log2 transformed and normalized by median subtraction. Bioinformatic analysis Pearson’s correlation heatmaps and hierarchical clustering were generated using the MeV software [53] . Protein profiles were grouped through a soft clustering approach ( Fig. 2 ), implemented in the GProx open source software package [54] . To this end, only proteins showing at least a fold change higher ±1 (in Log2 scale) compared with the 2°MEF in at least one time point were used ( Supplementary Data 2 ). Protein expression values were then standardized to have a mean value of zero and a standard deviation of one, ensuring that vectors of proteins with similar expression changes are close in Euclidean space. Clustering parameters such as Fuzzification, memberhip threshold and number of clusters were set at 1.45, 0.5 and 9, respectively. The protein members of each cluster were then subjected for functional analyses (that is, enrichment of GO terms, transcription factor binding and miRNAs prediction) using X2K software [55] . Statistical tests combining P value and z -score were used to detect overrepresentation of the annotations included in either GO, KEGG and CheA database. Transcription factor networks were created through the software TVNviewer [56] . Ingenuity Pathway Analysis was used to evaluate the enrichment of certain biological classes in protein with weak RNA to protein correlation. The processed proteomics data can be viewed alongside mRNA, miRNA, DNA methylation and histone mark analyses, on the same set of samples [38] , [39] , [40] , at www.stemformatics.org . This open-access resource allows collating, visualizing and analysing several large-scale data sets related to pluripotency. Pearson’s correlation heatmaps were generated using the MeV software. Functional analyses (that is, enrichment of GO terms, transcription factor binding) were done with the X2K software [55] . Statistical tests combining P value and z -score were used to detect overrepresentation of the annotations included in either GO, KEGG and CheA databases. Transcription factor networks were created with the software TVNviewer [56] . How to cite this article: Benevento, M. et al. Proteome adaptation in cell reprogramming proceeds via distinct transcriptional networks. Nat. Commun. 5:5613 doi: 10.1038/ncomms6613 (2014). Accession codes: Proteomics data have been deposited on Stemformatics ( www.stemformatics.org ) database and deposited to the ProteomeXchange Consortium ( http://proteomecentral.proteomexchange.org ) via the PRIDE partner repository (data set identifier PXD000413). The RNA-Seq data (data set identifier SRP046744) have been deposited to the NCBI Sequence Read Archive ( http://www.ncbi.nlm.nih.gov/sra ).